Annexin-A5 assembled into two-dimensional arrays promotes cell membrane repair Eukaryotic cells possess a universal repair machinery that ensures rapid resealing of plasma membrane disruptions. Before resealing, the torn membrane is submitted to considerable tension, which functions to expand the disruption. Here we show that annexin-A5 (AnxA5), a protein that self-assembles into two-dimensional (2D) arrays on membranes upon Ca 2+ activation, promotes membrane repair. Compared with wild-type mouse perivascular cells, AnxA5-null cells exhibit a severe membrane repair defect. Membrane repair in AnxA5-null cells is rescued by addition of AnxA5, which binds exclusively to disrupted membrane areas. In contrast, an AnxA5 mutant that lacks the ability of forming 2D arrays is unable to promote membrane repair. We propose that AnxA5 participates in a previously unrecognized step of the membrane repair process: triggered by the local influx of Ca 2+ , AnxA5 proteins bind to torn membrane edges and form a 2D array, which prevents wound expansion and promotes membrane resealing. Cells from many tissues, such as skeletal or cardiac muscle, skin, gut epithelium or vascular endothelium, are exposed to mechanical stress, which often induces the formation of tears in their plasma membranes [1] . Normal cells are able to repair these ruptures rapidly, whereas failure to reseal membranes leads to cell death and may contribute to the development of degenerative diseases, such as muscular dystrophies [2] . According to current models of cell membrane repair [1] , [3] , membrane resealing is an active process that requires extracellular Ca 2+ , intracellular vesicles and a step of Ca 2+ -dependent exocytosis [4] . Although small disruptions may reseal spontaneously in pure liposomes and erythrocyte membranes, the presence of a cortical cytoskeleton in cells creates considerable membrane tension, which prevents passive resealing [5] . Successful membrane resealing requires a decrease in membrane tension, which is achieved through vesicle exocytosis [6] , [7] or through the action of cytoskeleton depolymerizers [7] or surfactants [7] , [8] . For large membrane disruptions, the 'patch hypothesis' model proposes in addition that a membrane patch forms in the cytoplasm by homotypic fusion of intracellular vesicles before exocytotic fusion of the patch thus formed with the plasma membrane surrounding the disruption site [1] , [3] , [9] . Besides Ca 2+ and cytoplasmic vesicles, other components of the repair machinery start being identified. Dysferlin, a protein the gene mutations of which are responsible for muscular dystrophies [10] , has been shown to participate in the membrane fusion step of the repair process [11] , [12] , [13] . Another protein proposed to participate in membrane repair is MG53, a muscle-specific protein that becomes crosslinked when oxidants enter the cell through a disruption, and has recently been shown to interact with caveolin-3 and dysferlin [14] , [15] . Among other dysferlin-binding proteins, which include AHNAK, calveolin-3 and calpain-3 (ref. 2 ), two members of the annexin family, annexin-A1 (AnxA1) and A2 (AnxA2), have also been implicated in membrane repair [12] , [16] , although their roles remain to be elucidated [2] . Annexins form a family of soluble proteins that bind to membranes exposing negatively charged phospholipids, particularly phosphatidylserine (PS), in a Ca 2+ -dependent manner [17] . Annexins are formed by a four- (exceptionally eight-) fold repeat of 70 amino-acid domains that are highly conserved and by a variable amino (N)-terminal domain, which is assumed to be responsible for their functional specificities [18] . Following the determination of AnxA5 structure by Huber et al . [19] , atomic models have been obtained for several other annexins [20] . These structures show that annexins consist of a common membrane-binding core, which has the shape of a slightly curved rhomboid [19] with a convex membrane-binding face that presents Ca 2+ -binding loops and a concave face from which protrudes the N-terminal domain. The membrane-binding core is made of the cyclic arrangement of four α-helical domains, which correspond to the conserved sequence domains ( Fig. 1a ). Despite a wealth of studies describing the membrane-related properties of annexins, their biological functions remain largely unknown. Several reports have proposed intracellular functions for annexins, mainly AnxA2 in vesicle trafficking and membrane organization [17] . Paradoxically, although they lack a secretory signal peptide, annexins are found both intracellularly and extracellularly. Actually, the best-defined functions of the annexins concern extracellular AnxA1, AnxA2 and AnxA5, which possess anti-inflammatory [21] , pro-fibrinolytic [22] and anti-thrombotic [23] activities, respectively. A distinctive property of AnxA5 and several other annexins is to self-assemble into two-dimensional (2D) ordered arrays on membrane binding [17] , [24] , [25] , [26] , [27] , [28] , [29] , [30] , [31] , [32] . In the presence of mM Ca 2+ concentration, AnxA5 molecules bind to PS-containing membranes and self-assemble rapidly into trimers [33] , [34] , [35] and 2D ordered arrays of trimers [24] , [27] , [29] , [32] , [35] ( Fig. 1b ). Annexin arrays have been proposed to participate in the regulation of membrane organization and dynamics [17] , [35] and, in the case of AnxA5, to form an anticoagulant shield covering the surface of placental syncytiotrophoblasts [23] . 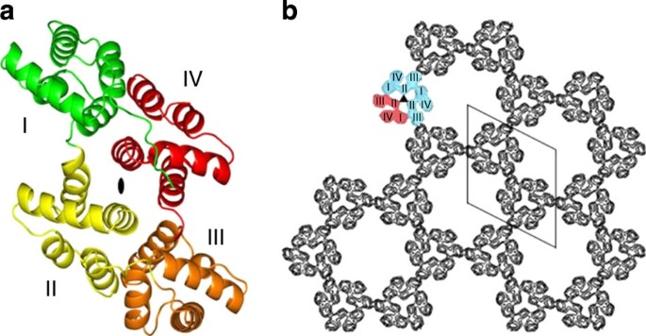Figure 1: Structure of soluble and membrane-bound AnxA5. (a) View of an AnxA5 molecule from the concave side of the molecule. AnxA5, the smallest annexin, is made up of four α-helical domains, numbered I–IV19, which form the conserved membrane-binding core of annexins. The molecule is observed along the pseudo twofold symmetry axis (dark ellipse), which relates module (I+IV) to module (II+III)19. This orientation corresponds almost to that of membrane-bound AnxA5 (refs27,58). This figure was created with PyMOL (http://pymol.org/) from PDB code 1AVR59. (b) Projection view of a 2D crystal of membrane-bound AnxA5 (adapted from ref.35). On membrane binding, AnxA5 molecules self-assemble into trimers and 2D crystals of trimers with various packing arrangements24,27,35. Panelbrepresents the main 2D crystalline arrangement formed by AnxA5 trimers, which has the symmetry of the two-sided plane group p6 (ref.35). A hexagonal unit cell is represented, with 17.7-nm unit cell side. An AnxA5 trimer is coloured, with one red and two blue monomers. Figure 1: Structure of soluble and membrane-bound AnxA5. ( a ) View of an AnxA5 molecule from the concave side of the molecule. AnxA5, the smallest annexin, is made up of four α-helical domains, numbered I–IV [19] , which form the conserved membrane-binding core of annexins. The molecule is observed along the pseudo twofold symmetry axis (dark ellipse), which relates module (I+IV) to module (II+III) [19] . This orientation corresponds almost to that of membrane-bound AnxA5 (refs [27] , [58] ). This figure was created with PyMOL ( http://pymol.org/ ) from PDB code 1AVR [59] . ( b ) Projection view of a 2D crystal of membrane-bound AnxA5 (adapted from ref. 35 ). On membrane binding, AnxA5 molecules self-assemble into trimers and 2D crystals of trimers with various packing arrangements [24] , [27] , [35] . Panel b represents the main 2D crystalline arrangement formed by AnxA5 trimers, which has the symmetry of the two-sided plane group p6 (ref. 35 ). A hexagonal unit cell is represented, with 17.7-nm unit cell side. An AnxA5 trimer is coloured, with one red and two blue monomers. Full size image The aim of the present study was to investigate whether AnxA5, and its 2D arrays, play a role in membrane repair. To address this question, we compared the responses to membrane injury of cells expressing AnxA5 to cells deficient in AnxA5 expression and investigated whether AnxA5 or a mutant of AnxA5 that is unable to form 2D arrays influenced membrane repair. Our results lead us to propose a novel model of membrane repair in which AnxA5 has a central role, promoting membrane resealing through the formation of 2D arrays at the level of membrane tears. Defect of membrane repair for AnxA5-null perivascular cells Membrane damage was applied to both mouse PV cells [36] , [37] , which express AnxA5 constitutively (wildtype (wt) PV), and to AnxA5-deficient PV cells in which the Anxa5 gene has been inactivated (AnxA5-null PV) [38] ( Supplementary Fig. S1 ). To induce membrane damage and assess membrane repair, cells were submitted to infrared laser irradiation in the presence of FM1-43 dye, following established procedures [11] . FM1-43 is a water-soluble dye, which becomes fluorescent on inserting into lipid membranes, yet is unable to cross membranes; therefore, cells with damaged plasma membrane exhibit an increase in fluorescence intensity due to the passive entrance of FM1-43 molecules in the cytosol and their incorporation into intracellular membranes. Irradiation conditions were first adjusted to the minimal power (160 mW) causing conspicuous membrane injury to most wt-PV cells, as indicated by an increase in cytoplasmic fluorescence intensity and the presence of a large, μm-size, disruption at the irradiation site ( Fig. 2a ). The kinetics of fluorescence intensity changes show that fluorescence intensity increases for ∼ 90 s, and then reaches a plateau ( Fig. 2b , filled circles). This stop in fluorescence increase indicates that cell membranes resealed, stopping further entrance of FM1-43. Membrane resealing correlates with the accumulation of vesicular lipid material near the disruption site ( Fig. 2a , frames 3–4). As Ca 2+ , at mM concentration, is required for membrane repair [4] , we performed control experiments in the presence of the Ca 2+ -chelating agent EGTA. With EGTA, wt-PV cells showed a continuous and large increase in fluorescence intensity ( Fig. 2c ; Supplementary Fig. S2a ), followed ultimately by cell death. This response is characteristic of the absence of membrane resealing. This preliminary set of results demonstrates that wt-PV cells possess a machinery that repairs membrane disruptions by means of a Ca 2+ -dependent mechanism involving the recruitment of intracellular vesicles to the site of membrane injury, in line with current knowledge on cell membrane repair [1] , [3] , [4] . 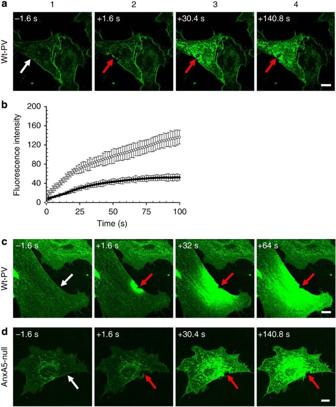Figure 2: Responses of wt-PV and AnxA5-null PV cells to 160-mW infrared irradiation. (a) Sequences of images showing the response of a wt-PV cell to 160-mW infrared irradiation in the presence of 2-mM Ca2+. In this panel, as well as in panelscandd, the area of membrane irradiation is marked with a white arrow before irradiation and a red arrow after irradiation. Image frames 1 and 2 were recorded 1.6 s before and 1.6 s after irradiation, respectively; frames 3–4 were recorded 30.4 and 140.8 s after irradiation, respectively, as indicated. (b) Kinetics of FM1-43 fluorescence intensity increase for wt-PV cells (filled circles) and AnxA5-null PV cells (empty circles) after membrane damage at 160-mW infrared irradiation in the presence of 2-mM Ca2+. Data represent the fluorescence intensity integrated over whole cell sections, averaged for 10 cells (±s.d.). For wt-PV cells, the fluorescence intensity reaches a plateau after∼90 s. For AnxA5-null PV cells, the fluorescence intensity increases continuously and is significantly larger than that for wt-PV cells, about ×3 larger at 100 s. (c) Sequence of images showing the response of a wt-PV cell to 160-mW infrared irradiation in the presence of 1-mM EGTA. Before irradiation, cells were washed three times in DPBS containing no CaCl2, then incubated in DPBS supplemented with 1-mM EGTA for 5 min. (d) Sequence of images showing the response of an AnxA5-null PV cell to 160-mW infrared irradiation in the presence of 2-mM Ca2+. Scale bars, 10 μm. Figure 2: Responses of wt-PV and AnxA5-null PV cells to 160-mW infrared irradiation. ( a ) Sequences of images showing the response of a wt-PV cell to 160-mW infrared irradiation in the presence of 2-mM Ca 2+ . In this panel, as well as in panels c and d , the area of membrane irradiation is marked with a white arrow before irradiation and a red arrow after irradiation. Image frames 1 and 2 were recorded 1.6 s before and 1.6 s after irradiation, respectively; frames 3–4 were recorded 30.4 and 140.8 s after irradiation, respectively, as indicated. ( b ) Kinetics of FM1-43 fluorescence intensity increase for wt-PV cells (filled circles) and AnxA5-null PV cells (empty circles) after membrane damage at 160-mW infrared irradiation in the presence of 2-mM Ca 2+ . Data represent the fluorescence intensity integrated over whole cell sections, averaged for 10 cells (±s.d.). For wt-PV cells, the fluorescence intensity reaches a plateau after ∼ 90 s. For AnxA5-null PV cells, the fluorescence intensity increases continuously and is significantly larger than that for wt-PV cells, about ×3 larger at 100 s. ( c ) Sequence of images showing the response of a wt-PV cell to 160-mW infrared irradiation in the presence of 1-mM EGTA. Before irradiation, cells were washed three times in DPBS containing no CaCl 2 , then incubated in DPBS supplemented with 1-mM EGTA for 5 min. ( d ) Sequence of images showing the response of an AnxA5-null PV cell to 160-mW infrared irradiation in the presence of 2-mM Ca 2+ . Scale bars, 10 μm. Full size image When AnxA5-null PV cells were submitted to the same irradiation conditions (160 mW) in the presence of Ca 2+ , their behaviour was similar to wt-PV cells in the absence of Ca 2+ , with a continuous entrance of FM1-43, followed by cell death ( Fig. 2d,b , open circles). This indicates that AnxA5-null PV cells present a defect in their membrane repair machinery. Rapid membrane repair of wt-PV cells submitted to low injury To gain further insight into these processes, we selected irradiation conditions for which wt-PV and AnxA5-null PV cells showed most distinct responses. At reduced laser intensity (80 mW), AnxA5-null PV cells responded as described above at 160 mW, with large membrane ruptures and absence of resealing ( Fig. 3a ; Supplementary Fig. S2b ). On the other hand, wt-PV cells presented two types of response. About 30% of wt-PV cells exhibited an increase of cytoplasmic fluorescence ( Fig. 3b ), which was significantly smaller (about ×3) than at 160 mW. Strikingly, none of these cells showed a macroscopic membrane rupture. We propose that the laser beam creates membrane microruptures, which allow the FM1-43 to enter, but are too small to be resolved. Most of wt-PV cells ( ∼ 70%) showed no detectable increase in cytoplasmic fluorescence ( Fig. 3c ). This indicates either that these cells were not damaged or, on the contrary, that membranes ruptured and rapidly repaired. The possibility that these cells were not properly irradiated is ruled out by the systematic observation of a complete photobleaching of FM1-43 dyes at irradiation sites (thin white arrow in Fig. 3c , frame 2; Supplementary Fig. S3 ). Therefore, we conclude that most wt-PV cells (about 70%) present a rapid resealing of membrane microruptures at reduced laser irradiation. 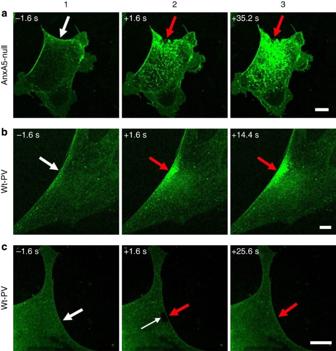Figure 3: Responses of wt-PV and AnxA5-null PV cells to 80-mW infrared irradiation. (a) Representative image series showing the response of an AnxA5-null PV cell to 80-mW infrared irradiation. The cell presents a macroscopic membrane rupture at the irradiated area and a large increase of cytoplasmic fluorescence intensity, as observed at 160 mW. (b,c) Image series showing two types of response for wt-PV cells irradiated at 80 mW. (b) A minor fraction (about 30%) of wt-PV cells presents an increase in cytoplasmic fluorescence intensity, yet no macroscopic membrane rupture. (c) The major fraction (about 70%) of wt-PV cells shows no increase in cytoplasmic fluorescence intensity. The areas of membrane irradiation are marked with a white arrow before irradiation and a red arrow after irradiation. Scale bars, 10 μm. Figure 3: Responses of wt-PV and AnxA5-null PV cells to 80-mW infrared irradiation. ( a ) Representative image series showing the response of an AnxA5-null PV cell to 80-mW infrared irradiation. The cell presents a macroscopic membrane rupture at the irradiated area and a large increase of cytoplasmic fluorescence intensity, as observed at 160 mW. ( b , c ) Image series showing two types of response for wt-PV cells irradiated at 80 mW. ( b ) A minor fraction (about 30%) of wt-PV cells presents an increase in cytoplasmic fluorescence intensity, yet no macroscopic membrane rupture. ( c ) The major fraction (about 70%) of wt-PV cells shows no increase in cytoplasmic fluorescence intensity. The areas of membrane irradiation are marked with a white arrow before irradiation and a red arrow after irradiation. Scale bars, 10 μm. Full size image The extracellular addition of AnxA5 promotes membrane repair Next, we tested whether the addition of extracellular AnxA5 had an effect on membrane repair. These experiments were motivated by the assumption that the differences exhibited by wt-PV and AnxA5-null PV cells were determined by the presence versus the absence of AnxA5 in these cells. In the presence of 1-μg ml −1 exogenous AnxA5, all wt-PV cells that were irradiated at 80 mW were characterized by a total absence of cytoplasmic fluorescence increase, which indicates that their membranes resealed rapidly ( Table 1 ). Even more striking, at 80 mW, was the fact that two-thirds of AnxA5-null PV cells presented also a rapid membrane resealing in the presence of 10-μg ml −1 AnxA5. At 160 mW, power at which 100% of both wt-PV and AnxA5-null PV cells presented macroscopic membrane ruptures in the absence of exogenous AnxA5, the addition of 10-μg ml −1 AnxA5 was sufficient to induce fast membrane repair for ∼ 85% wt-PV cells and 50% AnxA5-null PV cells, respectively. These results demonstrate that exogenous AnxA5 promotes membrane repair in AnxA5-expressing cells and restores repair ability in AnxA5-null PV cells. Therefore, AnxA5 has a central role in the membrane repair machinery. Table 1 Influence of the extracellular addition of AnxA5 and mtT-AnxA5 on cell membrane repair. Full size table AnxA5 binds exclusively to disrupted membrane areas Complementary experiments were performed to localize AnxA5 binding on infrared-damaged cells. Cy5-AnxA5 was found to bind exclusively to the sites of membrane injury, colocalizing with FM1-43 at initial stages after irradiation ( Fig. 4 ). Binding of Cy5-AnxA5 occurred very rapidly after damage, in the second range, with a total absence of binding before irradiation. The fact that AnxA5 binding remains limited to damaged membrane areas at later stages indicates further that PS-exposing membranes arise from membrane injury and not from apoptosis or necrosis, in which cases AnxA5 would cover the entire cell surface ( Supplementary Fig. S4 ). 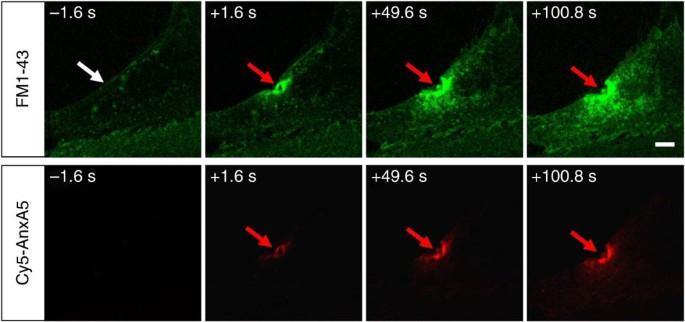Figure 4: Binding of Cy5-AnxA5 to injured membranes. Simultaneous recording of FM1-43 (top) and Cy5-AnxA5 (bottom) fluorescence of a wt-PV cell submitted to 160-mW infrared-induced membrane rupture. Cy5-AnxA5 binds exclusively at the level of the injured membrane, colocalizing initially with FM1-43 dyes. The area of membrane irradiation is marked with a white arrow before irradiation and a red arrow after irradiation. Scale bar, 10 μm. Figure 4: Binding of Cy5-AnxA5 to injured membranes. Simultaneous recording of FM1-43 (top) and Cy5-AnxA5 (bottom) fluorescence of a wt-PV cell submitted to 160-mW infrared-induced membrane rupture. Cy5-AnxA5 binds exclusively at the level of the injured membrane, colocalizing initially with FM1-43 dyes. The area of membrane irradiation is marked with a white arrow before irradiation and a red arrow after irradiation. Scale bar, 10 μm. Full size image The formation of AnxA5 2D arrays promotes membrane repair By which mechanism does AnxA5 promote cell membrane repair? The most remarkable in vitro property of AnxA5 is to self-assemble into trimers and 2D ordered arrays of trimers on PS-exposing membranes [29] , [35] ( Fig. 1b ). To investigate whether AnxA5 2D self-assembly had an influence on membrane repair, we produced AnxA5 mutants that lack the ability to form 2D arrays. The choice of the mutations was based on the fact that the monomer–monomer interface of AnxA5 trimers ( Fig. 5a ) presents several pairs of amino acids of opposite charges situated at distances close enough to form salt bridges [39] ( Fig. 5b ). In addition, Mo et al . [39] have shown that mutations of single amino acids were not sufficient to abolish the ability of AnxA5 to form trimers. Consequently, we produced multiple mutants in which several positively charged residues involved in salt bridging were replaced by negatively charged ones. The ability of AnxA5 mutants to form trimers was first assessed by transmission electron microscopy (TEM), according to established procedures [40] , [41] ( Supplementary Fig. S5 ). We found that all mutants with one, two or three mutations were still able to form 2D crystals, and thus trimers. Contrarily, all quadruple and quintuple mutants have lost the property of trimer and 2D crystal formation. The quintuple mutant mtT-AnxA5 (R16E, R23E, K27E, K56E, K191E) was selected for further analyses. To further ascertain that mtT-AnxA5 molecules are unable to form trimers, three-dimensional crystals of mtT-AnxA5 were grown in high Ca 2+ concentration and their structure was determined by X-ray crystallography. Indeed, all AnxA5 structures hitherto reported from three-dimensional crystals grown at high Ca 2+ concentration contain AnxA5 trimers, which are structurally homologous to membrane-bound trimers [39] , [42] , [43] . MtT-AnxA5 molecules crystallize in the P2 1 space group ( Supplementary Table S1 ; Supplementary Methods ) in which they pack as dimers with upside-down orientations ( Fig. 5c ). This result confirms that mtT-AnxA5 is unable to form trimers. 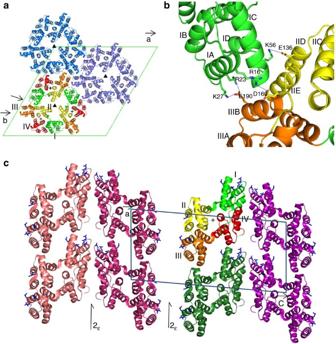Figure 5: Structure and packing of AnxA5 and mtT-AnxA5 in three-dimensional crystals. (a,b) Structure of trimers of recombinant rat AnxA5 (a) and monomer–monomer interface of a trimer (b) in R3 crystals (created from PDB code 1a8a)39,60. (a) The intramolecular pseudo twofold axes, which relate (I+IV) and (III+II) modules (indicated by crosses in each monomer of the bottom trimer) lie almost parallel (12°) to the threefold symmetry axes (black triangles) normal to the (a, b) plane. (b) Detailed structure of the monomer–monomer interface of an AnxA5 trimer, viewed along the arrow orientation in (a). A–E refer to AnxA5 α-helices, according to annexin nomenclature19. Several pairs of charged amino acids located at distances close enough to form salt bridges are indicated in ball-and-stick representation, with positively and negatively charged residues in blue and red, respectively. (c) Packing of mtT-AnxA5 molecules in high Ca2+content 3D crystals, along thebmonoclinic axis. MtT-AnxA5 molecules crystallize in the P21space group, with lattice parameters a=51.108 Å, b=67.184 Å, c=112.313 Å, β=94.79°. The asymmetric unit contains two protein molecules related by a non-crystallographic 2ɛscrew axis parallel to theaaxis, with a non-fractional pitch of ɛ=4.7 Å. The positions of two 2ɛscrew axes are indicated. MtT-AnxA5 molecules are oriented in thea, cplane with the intramolecular pseudo twofold axis (indicated by a cross in the AnxA5 monomer with I–IV numbering) lying almost normal (12°) to thea, cplane. This orientation is thus similar to that of native AnxA5 molecules shown inFigure 5a. Side chains of residues involved in salt-bridge interactions in AnxA5 trimers are shown as blue sticks. None of the residues participates in intermolecular contacts, with the exception of residue E16, which interacts through a Ca2+-mediated salt bridge with a neighbouring molecule along thebaxis. Figure 5: Structure and packing of AnxA5 and mtT-AnxA5 in three-dimensional crystals. ( a , b ) Structure of trimers of recombinant rat AnxA5 ( a ) and monomer–monomer interface of a trimer ( b ) in R3 crystals (created from PDB code 1a8a) [39] , [60] . ( a ) The intramolecular pseudo twofold axes, which relate (I+IV) and (III+II) modules (indicated by crosses in each monomer of the bottom trimer) lie almost parallel (12°) to the threefold symmetry axes (black triangles) normal to the (a, b) plane. ( b ) Detailed structure of the monomer–monomer interface of an AnxA5 trimer, viewed along the arrow orientation in ( a ). A–E refer to AnxA5 α-helices, according to annexin nomenclature [19] . Several pairs of charged amino acids located at distances close enough to form salt bridges are indicated in ball-and-stick representation, with positively and negatively charged residues in blue and red, respectively. ( c ) Packing of mtT-AnxA5 molecules in high Ca 2+ content 3D crystals, along the b monoclinic axis. MtT-AnxA5 molecules crystallize in the P2 1 space group, with lattice parameters a=51.108 Å, b=67.184 Å, c=112.313 Å, β=94.79°. The asymmetric unit contains two protein molecules related by a non-crystallographic 2 ɛ screw axis parallel to the a axis, with a non-fractional pitch of ɛ=4.7 Å. The positions of two 2 ɛ screw axes are indicated. MtT-AnxA5 molecules are oriented in the a, c plane with the intramolecular pseudo twofold axis (indicated by a cross in the AnxA5 monomer with I–IV numbering) lying almost normal (12°) to the a, c plane. This orientation is thus similar to that of native AnxA5 molecules shown in Figure 5a . Side chains of residues involved in salt-bridge interactions in AnxA5 trimers are shown as blue sticks. None of the residues participates in intermolecular contacts, with the exception of residue E16, which interacts through a Ca 2+ -mediated salt bridge with a neighbouring molecule along the b axis. Full size image Strikingly, unlike native AnxA5, mtT-AnxA5 was unable to promote membrane repair ( Table 1 ). We considered the possibility that the difference in behaviour between mtT-AnxA5 and native AnxA5 could be due to a difference in their membrane-binding properties, and measured their binding to PS-containing membranes. Native AnxA5 and mutant mtT-AnxA5 present undistinguishable binding characteristics to model membranes ( Fig. 6a ). This result is in agreement with previous indication that AnxA5–AnxA5 intermolecular interactions, in other words the formation of AnxA5 2D self-assemblies, does not contribute to membrane-binding affinity [44] . In addition, Cy5-mtT-AnxA5 bound to damaged membrane areas of irradiated wt-PV cells, similar to native AnxA5 ( Fig. 6b ). We conclude therefore that AnxA5 promotes membrane repair through the formation of ordered 2D arrays at the sites of membrane rupture. 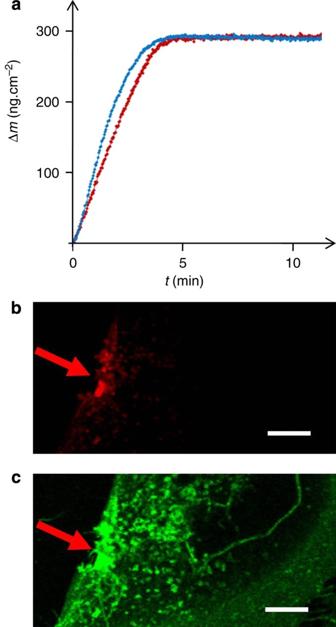Figure 6: Binding of mtT-AnxA5 to model membranes and infrared-injured cells. (a) Comparison of the binding of native AnxA5 (blue curve) and mtT-AnxA5 (red curve) to a supported lipid bilayer made of DOPC/DOPS (7:3, w/w), by QCM-D32. The formation of a supported lipid bilayer by deposition of small unilamellar vesicles on silica-coated quartz crystals takes place beforet=0 mn and is not shown here. Att=0 min, a solution of 5-μg ml−1AnxA5 or mtT-AnxA5 in HBS-Ca, pH 7.4, was injected at 150 μl min−1. The kinetics of adsorption and the adsorbed masses at saturation are almost identical for both proteins. The small difference observed between the kinetics of binding of native AnxA5 and mT-AnxA5 is equivalent to a difference in protein concentration of <1 μg ml−1, that is, 20% of nominal protein concentration, which is the level of accuracy of standard protein concentration assays. (b,c) Simultaneous recording of Cy5-mtT-AnxA5 (b) and FM1-43 (c) fluorescence of a wt-PV cell 1.6 s after 160-mW infrared-induced membrane rupture. The red arrows indicate the area of membrane irradiation. Scale bar, 10 μm. Figure 6: Binding of mtT-AnxA5 to model membranes and infrared-injured cells. ( a ) Comparison of the binding of native AnxA5 (blue curve) and mtT-AnxA5 (red curve) to a supported lipid bilayer made of DOPC/DOPS (7:3, w/w), by QCM-D [32] . The formation of a supported lipid bilayer by deposition of small unilamellar vesicles on silica-coated quartz crystals takes place before t =0 mn and is not shown here. At t =0 min, a solution of 5-μg ml −1 AnxA5 or mtT-AnxA5 in HBS-Ca, pH 7.4, was injected at 150 μl min −1 . The kinetics of adsorption and the adsorbed masses at saturation are almost identical for both proteins. The small difference observed between the kinetics of binding of native AnxA5 and mT-AnxA5 is equivalent to a difference in protein concentration of <1 μg ml −1 , that is, 20% of nominal protein concentration, which is the level of accuracy of standard protein concentration assays. ( b , c ) Simultaneous recording of Cy5-mtT-AnxA5 ( b ) and FM1-43 ( c ) fluorescence of a wt-PV cell 1.6 s after 160-mW infrared-induced membrane rupture. The red arrows indicate the area of membrane irradiation. Scale bar, 10 μm. Full size image According to current models, membrane resealing is an active process that requires extracellular Ca 2+ , intracellular vesicles and a step of Ca 2+ -dependent exocytosis [1] , [3] , [4] , [9] . We propose that immediately after membrane rupture ( Fig. 7a,b ), AnxA5 participates in a previously unrecognized step of the repair process ( Fig. 7c,d ), which is followed by the membrane fusion events ( Fig. 7e ). Membrane ruptures create microenvironments in which extracellular and intracellular components mix; in particular, the high intracellular concentrations of PS and AnxA5 mix with the high extracellular concentration of Ca 2+ . Triggered by the local increase in Ca 2+ concentration, AnxA5 binds to PS molecules exposed at the edges of torn membranes at which it self-assembles into 2D arrays. In vitro studies have indicated that AnxA5 2D arrays rigidify lipid monolayers and reduce the lateral diffusion of phospholipids [45] , [46] . We propose that the formation of AnxA5 2D array at a ruptured membrane strengthens the membrane and prevents the expansion of the tear. By counteracting membrane tension due to cytoskeleton attachment, AnxA5 2D arrays promote membrane resealing in a way similar to that of other agents that lower membrane tension, similar to cytoskeleton depolymerizers [7] or surfactants [7] , [8] . 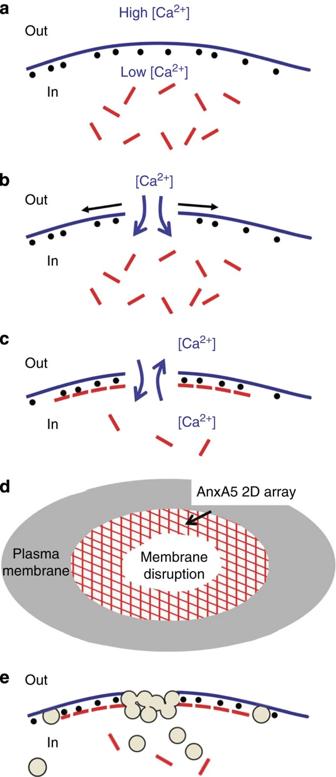Figure 7: Model of cell membrane repair. (a) Intact cell membrane. The extracellular (Out) and intracellular (In) milieus differ by their high versus low Ca2+concentrations, and the absence versus presence of AnxA5 (red rods) and PS (black spheres), respectively. (b) Local rupture of a cell membrane. Forces resulting from membrane tension tend to expand the tear laterally (black arrows). (c) The formation of an AnxA5 2D array at the torn membrane stops wound expansion. On membrane rupture, a microenvironment is formed in which the intracellular and extracellular milieus mix, providing optimal conditions for the formation of tight complexes between Ca2+, PS and AnxA5 (ref.44). AnxA5 molecules bind to PS molecules exposed at ruptured membrane edges, form trimers and 2D arrays. These AnxA5 2D self-assemblies stabilize the membrane and stop expansion of the tear. (d) Top view of a membrane disruption with an AnxA5 2D array surrounding the tear. (e) Membrane resealing. Cytoplasmic vesicles are recruited at the ruptured membrane area and fuse by exocytosis with the plasma membrane, either directly as single vesicles or as a patch formed by homotypic fusion of intracellular vesicles1,9. The resulting increase in membrane surface and decrease in membrane tension lead to membrane resealing. Figure 7: Model of cell membrane repair. ( a ) Intact cell membrane. The extracellular (Out) and intracellular (In) milieus differ by their high versus low Ca 2+ concentrations, and the absence versus presence of AnxA5 (red rods) and PS (black spheres), respectively. ( b ) Local rupture of a cell membrane. Forces resulting from membrane tension tend to expand the tear laterally (black arrows). ( c ) The formation of an AnxA5 2D array at the torn membrane stops wound expansion. On membrane rupture, a microenvironment is formed in which the intracellular and extracellular milieus mix, providing optimal conditions for the formation of tight complexes between Ca 2+ , PS and AnxA5 (ref. 44 ). AnxA5 molecules bind to PS molecules exposed at ruptured membrane edges, form trimers and 2D arrays. These AnxA5 2D self-assemblies stabilize the membrane and stop expansion of the tear. ( d ) Top view of a membrane disruption with an AnxA5 2D array surrounding the tear. ( e ) Membrane resealing. Cytoplasmic vesicles are recruited at the ruptured membrane area and fuse by exocytosis with the plasma membrane, either directly as single vesicles or as a patch formed by homotypic fusion of intracellular vesicles [1] , [9] . The resulting increase in membrane surface and decrease in membrane tension lead to membrane resealing. Full size image The hypothesis that cell membrane rupture enables the local and transient mixing of extracellular and intracellular compartments, hitherto poorly appreciated, offers a simple explanation for the long-debated question of the extracellular presence of annexins, which may apply to other proteins that also lack a secretory signal sequence. The fact that all annexins bind to PS-exposing membranes, some of them at lower Ca 2+ concentration than AnxA5 (ref. 47 ), raises the question of competition for membrane surface between annexins. We show here that AnxA5 binds rapidly to PS-exposing injured membranes ( Fig. 4 ). The high PS concentration of the plasma membrane inner leaflet [48] , [49] may allow simultaneous binding of annexins. On the other hand, AnxA5 2D arrays present an open structure, in the sense that AnxA5 proteins occupy only ∼ 65% of the crystal surface. Protein-free spaces large enough to accommodate additional AnxA5 trimers are present at the sixfold symmetry centres [29] ( Supplementary Fig. S6 ). It is therefore likely that other annexins, as well as other integral or peripheral membrane proteins, can be integrated within AnxA5 2D arrays, and may thus colocalize with AnxA5 at injured membrane areas. This hypothesis is supported by a recent study from Skrahina et al . [47] who showed that AnxA5 forms heterogenous assemblies with AnxA1 or AnxA2 on plasma membranes of ionomycin-treated cells and speculated that such assemblies participate in membrane repair. The finding that AnxA5 promotes membrane repair allows us to speculate on a collective role of annexins in protecting cells against membrane damage effects. The anti-inflammatory, pro-fibrinolytic and anti-thrombotic activities of AnxA1 (ref. 21 ), AnxA2 (ref. 22 ) and AnxA5 (ref. 23 ), respectively, can indeed be understood in the context of a global machinery protecting cells against damages resulting from membrane rupture. In the absence of such a protective mechanism, the release of cytoplasmic material outside the cell through a membrane tear would initiate an inflammatory reaction, and the exposure of PS molecules to the blood compartment would initiate a coagulation process ending up with fibrin formation. It is likely that cells have developed mechanisms protecting them against such undesired effects. It is thus striking that the described functions of AnxA1, AnxA2 and AnxA5 correspond to such protection activities. Annexins may also participate in other aspects of the membrane repair machinery, for example, in the transport of cytoplasmic vesicles along actin filaments [50] or in the step of vesicle aggregation preceding fusion events [51] , [28] . Another possibility is that different annexins bind at different Ca 2+ concentrations to sites of different lipid compositions [52] , [53] . Therefore, we speculate that, together with Ca 2+ , annexins form an emergency team that orchestrates the cell membrane repair machinery and protects cells against the direct and collateral effects of plasma membrane rupture. Given the vital importance of AnxA5 function for cells, it will be interesting to investigate whether AnxA5 may be of therapeutic value in diseases or pathologies associated with defects in the membrane repair machinery. Isolation and culture of perivascular cells Populations of PV cells were isolated from adult-brain meninges of 4- to 6-month-old mice after digestion with collagenase, trypsin and DNA seI [36] , [37] . AnxA5-null PV cells and AnxA5-expressing wt-PV cells were isolated from Anxa5 LacZ/LacZ and Anxa5 LacZ/+ mice, respectively ( Supplementary Fig. S1 ). Single-cell suspensions were vitally stained for β-galactosidase activity by fluorescein-di-β- D -galactopyranoside and viable fluorescein-positive cells were sorted by fluorescence-activated cell sorting (MoFlow, Cytomation). Cells were expanded in MesenCult medium according to the supplier's protocol (Stemcell Technologies). Genotypes were confirmed by PCR [38] . Established cell lines were maintained in DMEM supplemented with 10% fetal bovine serum, 5-mM L -glutamine, 100 U ml −1 penicillin and 100-μg ml −1 streptomycin, at 37 °C in a 5% CO 2 incubator. Membrane rupture and repair assays Cells (2×10 4 cells per cm 2 ) were cultivated in complete DMEM without red phenol on eight-well Lab-Tek plates (Nalge Nunc International) one day before the experiment. Fluorescence imaging was performed on a TCS SP2 AOBS Leica confocal scanning microscope with an HCX-PL-APO-CS 63.0×1.40 oil objective lens. Before live-cell imaging, cells were washed three times in Dulbecco's phosphate buffer saline (DPBS) containing 0.9-mM CaCl 2 (DPBS-Ca 2+ ), incubated for 5 min in DPBS-Ca 2+ supplemented with 5-μg ml −1 FM1-43FX (further referred to as FM1-43) and maintained over ice until imaging. FM1-43 was excited by the 488-nm laser line (intensity set at 30% maximal power) and fluorescence emission was measured between 500 nm and 570 nm. Images (512×512 pixels; 119×119 μm full size) were acquired at 1.6-s intervals with pinhole set to 1 Airy unit. To induce membrane damage, cells were irradiated at 820 nm with a Chameleon-Vision mode-locked Titanium:Sapphire laser (Coherent). Irradiation consisted of three successive scans, of 1.6 s each, of a 3×3-μm area with a power of either 80 mW or 160 mW. A thorough focusing protocol was applied to ensure optimal and reproducible conditions of irradiation. First, focusing was adjusted by maximizing the fluorescence intensity of FM1-43 at the plasma membrane. Second, the three successive images of the 3×3-μm irradiated areas were analysed to verify that FM1-43 dyes were totally photobleached during irradiation ( Supplementary Fig. S3 ). Only image series showing complete FM1-43 photobleaching were selected for this study. Membrane rupture and repair processes were monitored by recording FM1-43 fluorescence images. For quantitative analysis, the fluorescence intensity was integrated over whole cell sections and corrected for the fluorescence value measured before irradiation, using ImageJ program. Fluorescence imaging was carried out at 25 °C. Production of AnxA5 and AnxA5 mutants Recombinant rat AnxA5 was expressed in Escherichia coli BL21(DE3) cells and purified by Superdex-75 (GE-Healthcare) size-exclusion chromatography, followed by MonoQ HR5/5 (GE-Healthcare) anion-exchange chromatography [54] . A series of AnxA5 mutants was produced using standard methods of site-directed mutagenesis [55] . Five AnxA5 single mutants were produced, corresponding to the mutations R16E, R23E, K27E, K56E and K191E, by replacing the AGG, CGG, AAA, AAG and AAG codons by a GAG codon for R16E, R23E, K27E, K56E and K191E, respectively. The following double, triple, quadruple and quintuple mutants were produced: K27E/K191E, R16E/K27E/K191E, R23E/K27E/K191E, R16E/K27E/K56E, R16E/R23E/K27E/K191E, R16E/K27E/K56E/K191E and R16E/R23E/K27E/K56E/K191E. Mutations were verified by double-strand DNA sequence analysis. Proteins were expressed and purified as indicated above for AnxA5. Production of Cy5-AnxA5 A double mutant (C314S, T163C) AnxA5, referred to as AnxA5-SH, was produced and purified as follows. To construct AnxA5-SH protein, the only cysteine present in wt-AnxA5 was replaced by a serine (C314S) and a single cysteine was introduced at position 163 (T163C), in a highly exposed region on the concave face of the protein opposite to its membrane-binding face. AnxA5-S-S-Anx5 dimers were produced by oxidation of Anx5-SH and purified by MonoQ HR5/5 anion-exchange chromatography [54] . Cy5-AnxA5 was synthesized by covalent coupling of Cy5-N-ethylmaleimide to AnxA5-SH as follows. The desired amount of AnxA5-S-S-AnxA5 dimer (0.2 μmole in 17.6 ml of 250-mM NaCl, 20-mM Tris, pH 8.0) was reacted with TCEP (8.8 μmol in a HEPES-buffered saline (HBS) prepared from 10-mM HEPES, 150-mM NaCl and 2-mM NaN 3 at pH 7.4) for 30 min at room temperature. Reduced AnxA5-SH was mixed with a threefold excess of Cy5-N-ethylmaleimide and incubated for 3 h at ambient temperature in obscurity. Cy5-AnxA5 was separated from non-reacted Cy5-N-ethylmaleimide by ultrafiltration, using an Amicon ultrafiltration cell (Millipore) and 10-kDa MWCO membranes. After four rinses with 10 ml of 20-mM Tris, pH 8.0, Cy5-AnxA5 was further purified by MonoQ HR5/5 anion-exchange chromatography. A yield of 4.2-mg pure Cy5-Anx5 was obtained, corresponding to an overall yield of ∼ 30%. Stock solutions of 1-mg ml −1 Cy5-AnxA5 were stored at 4 °C. Localization of Cy5-AnxA5 binding on wt-PV cells Cy5-labelled AnxA5 and mtT-AnxA5 proteins were used for localizing AnxA5 binding on irradiated wt-PV cells. Cells were incubated in the presence of 5-μg ml −1 FM1-43 and 3-μg ml −1 Cy5-AnxA5 for 5 min before irradiation. Cy5-Anx5 was excited by the 633-nm laser line (intensity set at 60% maximal power) and its emission recorded between 650 and 750 nm. Two-Dimensional crystallization of AnxA5 proteins on lipid monolayers The ability of AnxA5 mutants to form 2D crystals on PS-containing membranes was investigated by the method of protein crystallization on lipid monolayers, as described in ref. 40 . Briefly, a lipid monolayer was formed by applying 0.6 μl of a lipid mixture containing 450-μM 1,2-dioleoyl- sn -glycero-3-phosphocholine (DOPC) and 150-μM 1,2-dioleoyl- sn -glycero-3-[phospho-L-serine] (DOPS) dissolved in chloroform:hexane (1:1, v:v) over a 17-μl droplet containing 100-μg ml −1 AnxA5 or AnxA5 mutant in HBS supplemented with 2-mM CaCl 2 (HBS-Ca) at pH 7.4. After 1-h incubation at ambient temperature, the lipid–protein monolayer present at the air–water interface was transferred onto a perforated carbon-coated 200-mesh copper grid (Ted Pella) by horizontal lifting. The grid was rinsed with water, negatively stained with 1% uranyl acetate and coated with a thin layer of carbon to increase stability. TEM observations were performed with a CM-120 FEI microscope operated at 120 kV. Images were recorded under minimal dose conditions on a 2×2k USC-1000 slow-scan CCD camera (Gatan) at a nominal magnification of ×45,000. Fourier transforms of TEM images were calculated using Gatan-Digital Micrograph software. The presence of 2D crystals was assessed by direct observation of the Fourier transforms. Binding of AnxA5 proteins to lipid bilayers by QCM-D Binding of AnxA5 and mtT-AnxA5 to PS-containing supported lipid bilayers was measured by Quartz Crystal Microbalance with Dissipation monitoring (QCM-D) with a Q-SENSE E4 system (Q-SENSE) [32] . Changes in resonance frequency, Δ f , and in dissipation, Δ D , were measured at several harmonics (15, 25, 35 MHz) simultaneously. Adsorbed masses, Δ m , were calculated according to the Sauerbrey equation, Δm=– C· Δ f norm , with the mass sensitivity constant C =17.7 ng cm –2 Hz –1 and Δ f norm =Δ f n / n , with n being the overtone number [56] . A supported lipid bilayer was formed on a silica-coated quartz crystal by deposition of small lipid vesicles made of DOPC/DOPS (7:3, w:w) [56] , [57] . After a stable lipid bilayer was formed on the quartz crystal, as indicated by characteristic values of 25 Hz and <0.2×10 −6 for Δ f and Δ D , respectively [57] , the chamber was rinsed with HBS-Ca, pH 7.4, to remove the excess lipid vesicles. Protein solutions were injected at 5 μg ml −1 and a flow rate of 150 μl min −1 , and adsorption was measured by recording Δ f and Δ D changes. In Figure 6a , Δ m values corresponding to the fifth harmonics ( n =5, that is, 25 MHz) are presented. The changes in dissipation Δ D are not presented because the monolayers formed by AnxA5 are rigid and present a negligible increase in Δ D [32] . Accession codes: Atomic coordinates and structure factor amplitudes of mtT-AnxA5 have been deposited to the RCSB Protein Data Bank with entry code 2h0k How to cite this article: Bouter, A et al . Annexin-A5 assembled into two-dimensional arrays promotes cell membrane repair. Nat. Commun. 2:270 doi: 10.1038/ncomms1270 (2011).